A one-dimensional optomechanical crystal with a complete phononic band gap Recent years have witnessed the boom of cavity optomechanics, which exploits the confinement and coupling of optical and mechanical waves at the nanoscale. Among their physical implementations, optomechanical (OM) crystals built on semiconductor slabs enable the integration and manipulation of multiple OM elements in a single chip and provide gigahertz phonons suitable for coherent phonon manipulation. Different demonstrations of coupling of infrared photons and gigahertz phonons in cavities created by inserting defects on OM crystals have been performed. However, the considered structures do not show a complete phononic bandgap, which should enable longer lifetimes, as acoustic leakage is minimized. Here we demonstrate the excitation of acoustic modes in a one-dimensional OM crystal properly designed to display a full phononic bandgap for acoustic modes at 4 GHz. The modes inside the complete bandgap are designed to have high-mechanical Q-factors, limit clamping losses and be invariant to fabrication imperfections. Optomechanical (OM) coupling, the direct interaction of electromagnetic radiation and mechanical vibrations of matter, can be greatly enhanced by confining electromagnetic radiation in a cavity. As the establishment of cavity optomechanics [1] , [2] , [3] , the transduction of phonons through light has led to a wide variety of applications in sensing [4] , [5] , [6] and communications [7] , [8] , [9] , [10] . Moreover, the manipulation of mechanical degrees of freedom with light, with reported demonstrations of energy transfer from photons to phonons (amplification [11] ) and from phonons to photons (sideband resolved OM cooling [12] , [13] ), has paved the way towards the coherent quantum control of a mechanical oscillator [14] , [15] , [16] , [17] , [18] . The recent experimental demonstration of a mechanical resonator being cooled down to the ground state [19] , [20] with less than a single confined phonon (on average), and coherent effects like optomechanically induced transparency [21] , [22] and coherent coupling in the well-resolved sideband regime (OM normal mode splitting [23] ), together confirm OM cavities as ideal building blocks for phonon-based quantum computation. However, the conditions that a cavity OM system, which range from the macroscopic to the atomic domain and make use of radiation covering the microwave to the visible domain [24] , must fulfil to allow phonon coherent manipulation are strongly restrictive. The OM vacuum coupling ( g ) strength is one of the key factors, with the highest reports giving g/ 2π rates in the MHz range [4] , [25] , [26] , [27] . This g factor multiplied by the photon lifetime in the cavity ( τ cav ) gives an important figure of merit ( g / κ , where κ is the optical cavity decay rate, κ =1/ τ cav ), which can be related with the interaction strength per photon inside the cavity. Ground state cooling (that is, average phonon population <1 at the ground state) requires that the OM system be within the side-band-resolved limit. In other words, the mechanical oscillation period must be less than the lifetime in the cavity ( T mec < τ cav ). In addition, it is important to preserve the phonon mode from the interaction with thermally populated acoustic phonons, a decay channel that limits the coherence time of the system. High-frequency phononic modes ( ω m in the GHz) are less populated for the same temperature ( n th ≈ k B T th / ħω m ), and can be cooled down to the ground state even without OM-assisted cooling [28] . The quality of the mechanical cavity ( Q mec ) is a signature of the level of isolation reached in the phonon confinement. A good figure of merit for quantum-coherent phonon manipulation is Q mec · ω m /2π. Goryachev et al. [29] reached 7.8 × 10 16 Hz using a microwave system, whereas Chan et al. [20] reached 3.9 × 10 14 Hz with an OM crystal. OM crystals [30] , [31] , [32] are simultaneously photonic and phononic crystals that confine in the same structure photons and phonons, so that when engineered properly they can lead to strong photon–phonon interaction. OM crystals offer a practical advantage over other OM systems: they can be easily integrated in chip platforms, which enable the design of multiple OM elements as circuits. However, they have also an edge on the fundamental physical limits attainable in phonon isolation, as their typical phonon frequency lies in the high GHz range and phononic band gaps can be designed to prevent phonon propagation at certain frequency ranges. A complete phononic band gap is defined by the absence of any phononic band in a given frequency range, meanwhile, a pseudo-band gap is defined by the absence of bands of a particular symmetry in the frequency range of definition, even if there are still bands of other symmetries at that frequencies. In Chan et al. [20] , [26] , unwanted imperfections during fabrication can break the perfect symmetry of the ideal (designed) structure and allow coupling among different symmetry phononic propagative bands inside the pseudo-bandgaps. This loss mechanism can be cancelled out by surrounding the structure with a phononic radiation shield (a two-dimensional phononic crystal with a complete band gap) that prohibits the existence of leaking modes. This shield could be integrated in the nanobeam mirror cells; however, in practice, the design of a one-dimensional (1D) cavity that is simultaneously photonic and phononic is even more restrictive and to date, has not yet been accomplished. Limiting the losses increases the phonon lifetime and should enable multiple coherent phonon operations in a quantum-computing scheme that is based on phonons and controlled (or read out) by light. Safavi-Naeini et al. [33] very recently demonstrated that use of a full phononic bandgap is essential to reduce clamping losses in a two-dimensional OM crystal. In this paper, we present a 1D silicon OM crystal built up so that it displays a dual absolute band gap for both phonons and photons [34] , as proposed by Maldovan and Thomas in ref. 35 . This type of structure has been named a phoXonic crystal [36] . The key advantage of the unit cell that we use over previous approaches is that optical properties are mainly determined by the inner beam width and the hole size and spacing, whereas the mechanical properties are specially affected by the stub width and size. Such an approach effectively uncouples the design of the optical and the mechanical cavities, thereby enabling a full 1D phononic band gap for propagating modes and a photonic bandgap for TE-like (Transverse Electric even parity) optical modes. 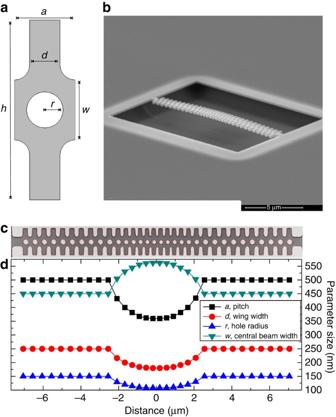Figure 1: The 1D silicon OM crystal with a full phononic bandgap. (a) Ideal unit cell with its defining parameters shown (adapted from ref.34). (b) Tilted SEM image of typical fabricated device. (c) SEM image of the fabricated OM cavity with dimensions corresponding (1:1) to the ordinate axis. The red trace in the SEM image corresponds to the profile used in the FEM calculations to model the real structure. (d) Plots of parameter variation to build the OM defect crystal cavity. Device design Figure 1a sketches the top view of the unit cell of the proposed OM crystal, a 220-nm-thick nanobeam. The cavity is built by varying in a parabolic way towards the centre of the structure the cell width ( a , pitch), hole radius ( r ) and stub width ( d ) the same percentage (percentage of reduction (PR)), meanwhile the beam width ( w ) is increased towards the centre. In the OM cavity presented in Fig. 1b , PR is 72%. These and other parameters (for example, hole to ellipse and stub shape) could be varied in an independent way at the expense of a numerically complex optimization process [26] , which suggest pending areas for improvement in the OM coupling. On top of the graph, we present a scanning electron microscope (SEM) image of the OM cavity discussed onwards. The fabrication imperfections are taken into account in the simulations along the paper (see Methods ‘Fabrication imperfections’). We have plotted in red the contour of the structure obtained from the SEM image trace. This contour is used to calculate the optical and mechanical properties of the structure using finite element method (FEM) in commercial software Comsol. We use 10 mirror cells at every side of the cavity, composed by 12 cells, and centred in a beam connector. Figure 1: The 1D silicon OM crystal with a full phononic bandgap. ( a ) Ideal unit cell with its defining parameters shown (adapted from ref. 34 ). ( b ) Tilted SEM image of typical fabricated device. ( c ) SEM image of the fabricated OM cavity with dimensions corresponding (1:1) to the ordinate axis. The red trace in the SEM image corresponds to the profile used in the FEM calculations to model the real structure. ( d ) Plots of parameter variation to build the OM defect crystal cavity. Full size image Optical properties The photonic band diagram ( Fig. 2a ) of the OM cavity’s mirror cells presents a band gap for TE modes. The variation of the cell towards the centre of the OM cavity creates an effective confining potential by pulling up the modes of the second and third TE band up from the X point. The tapering allows us achieving strongly confined, high-Q photonic modes at telecom wavelengths. We place a tapered fibre loop (see ‘Experimental methods’) close to the device standing partially on the frame around the substrate. In all the experiments, light is coupled in and out of the device from the tapered fibre. A Lorentzian fit to the experimental results for the fabricated structure ( Fig. 2b ) shows an optical Q-factor of 1.06 × 10 4 and a power drop of 43% for the mode at 1,529 nm. The total cavity decay rate κ /2π is 18.4 GHz assuming bidirectional coupling to the tapered fibre, with an intrinsic decay rate κ i /2π of 13.9 GHz and an extrinsic decay rate κ e /2π of 4.52 GHz. We identified six confined optical modes in the wavelength range between 1,470 and 1,600 nm by comparing the simulations and the experimental results. 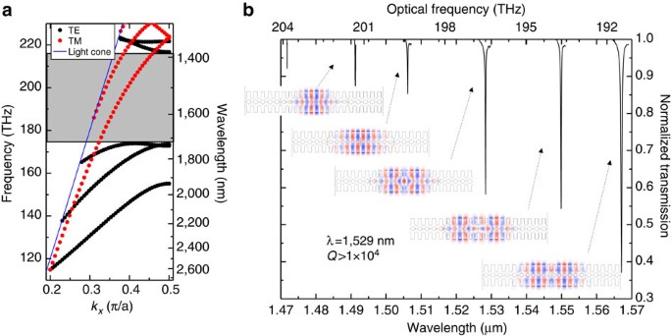Figure 2: Photonic properties of the OM nanobeam crystal. (a) Photonic band diagram of an idealized mirror cell, showing the TE optical modes (black plots), the Transverse Magnetic (TM) modes (red dots) and the pseudo bandgap for the TE mode (grey area). (b) Experimental optical spectroscopy curve of device 1, with FEM simulations of an idealized device shown for reference. Figure 2: Photonic properties of the OM nanobeam crystal. ( a ) Photonic band diagram of an idealized mirror cell, showing the TE optical modes (black plots), the Transverse Magnetic (TM) modes (red dots) and the pseudo bandgap for the TE mode (grey area). ( b ) Experimental optical spectroscopy curve of device 1, with FEM simulations of an idealized device shown for reference. Full size image Mechanical properties By adjusting the detuning between the laser and the cavity in the blue sideband, we maximize the transduction for a fixed low laser power. The power drop is limited to 4.5 μW, with a detuning value of Δ =κ /2, so we have less than 1,000 photons in the cavity ( Fig. 3a , top). We should expect to transduce only modes symmetric to the planes normal to the nanobeam (symmetric/symmetric) but fabrication imperfections break and mix the symmetries. By comparing FEM simulations and the Radio Frequency (RF) spectrum, we have identified five different phononic mode families. Exemplary displacement profiles are shown in Fig. 3a top, where they are linked (with arrows) to the corresponding experimental transduced modes. We confirm the grouping of the phononic modes observed by changing the minimum reduction percentage of the parabolic defect (hundreds of devices fabricated, simulated and characterized) and the optical mode used to transduce them. The values of the mechanical Q -factors measured at room temperature and atmospheric pressure are ca 2,000. We achieve amplification of phononic modes from families at 5.5 and 7 GHz by measuring in coupling conditions within the resolved band limit ( Supplementary Methods and Supplementary Figure 6 ). 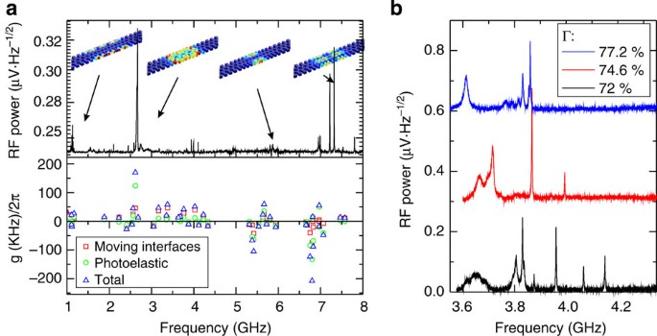Figure 3: Phononic properties of the OM nanobeam crystal. (a) Top, RF spectrum of the phononic modes transduced by the device, showing FEM simulations of an idealized (as designed) structure. We have identified five different families (four are plotted here; the fifth one can be observed inFig. 4). Bottom, vacuum OM coupling (g) calculations corresponding to the fabricated OM cavity ofFigs 1and2(limited to those 50 phonon modes with the highestg). We distinguish between contributions of the moving interfaces effects (red hollow square) and the photoelastic effects (green hollow circle). The total OM coupling is the addition of both contributions (blue hollow triangle). (b) Experimental RF spectra of a different series of OM cavities, whereby the deepness of the defect (1-PR) is increased. The confined modes shift towards higher frequency entering into the complete band gap. Figure 3: Phononic properties of the OM nanobeam crystal. ( a ) Top, RF spectrum of the phononic modes transduced by the device, showing FEM simulations of an idealized (as designed) structure. We have identified five different families (four are plotted here; the fifth one can be observed in Fig. 4 ). Bottom, vacuum OM coupling ( g ) calculations corresponding to the fabricated OM cavity of Figs 1 and 2 (limited to those 50 phonon modes with the highest g ). We distinguish between contributions of the moving interfaces effects (red hollow square) and the photoelastic effects (green hollow circle). The total OM coupling is the addition of both contributions (blue hollow triangle). ( b ) Experimental RF spectra of a different series of OM cavities, whereby the deepness of the defect (1-PR) is increased. The confined modes shift towards higher frequency entering into the complete band gap. Full size image In Fig. 3a , we plot the vacuum OM coupling rate split in moving interfaces and photoelastic contributions for the modes confined in the cavity. The maximum absolute rates calculated are in the hundreds of KHz range for the modes at 2.61 GHz ( g /2π=168 kHz) and 6.8 GHz ( g /2π=−206 kHz), comparable to previous reports in OM crystal cavities and confirmed experimentally for some of the modes ( Supplementary Methods and Supplementary Figs 4 and 5 ). Moreover, in most of the cases, the contributions of the moving interface and the photoelastic effects are additive, what is a remarkable particularity of the geometry proposed that makes it extremely interesting. The optimization process becomes more promising in this case, as up to now, the maximum OM coupling rates are obtained by maximizing the dominance of one of these effects over the other one, rather than by maximizing both of them simultaneously. The origin of the observed families can be linked directly to the phononic bands that we used to create them. In Fig. 4a , we plot in the central panel the phononic band diagram for an idealized (without fabrication imperfections; black dots) and all real mirror cells (grey dots). The red dots in the same panel draw the symmetric/symmetric bands that should theoretically lead to OM coupling. At the side panels, we plot the confinement potentials created by the modification of the cells towards the centre. These confinement potentials correspond perfectly with the confined modes simulated and measured in Fig. 3 . The modes around 4 and 5.5 and above 7 GHz are drawn from the X point ( k x =π /a ), the origin of the stronger modes at 1 and 2.5 GHz is the Γ point ( k x =0). The dispersion created by unwanted fabrication imperfections breaks the symmetry and allows mode coupling between modes of different symmetries, breaking the effectiveness of the mode isolation in pseudo-bandgaps (green rectangles). Nevertheless, the modes inside the complete bandgap (light blue) should be immune to such effects, as shown by simulations (FEM simulations of Fig. 4b , see Supplementary Figure 8 ). The mechanical Q-factor increases up to 7 × 10 7 for the mode placed deeper in the bandgap, even if the fabrication imperfections limit it strongly. The fabricated device presents attenuation of the transmitted signals of at least eight orders of magnitude for the zone surrounding the bandgap as simulated in the inset of Fig. 4b . A fair agreement between simulations and measurements allows us to label the measured modes and identify three of them as confined inside the complete bandgap. In Fig. 3b , we show how by increasing the deepness of the defect in the OM cavity (1-PR), the confined modes around the low-frequency band edge of the complete bandgap can be displaced into it by increasing their frequency (see Supplementary Figure 7 ). 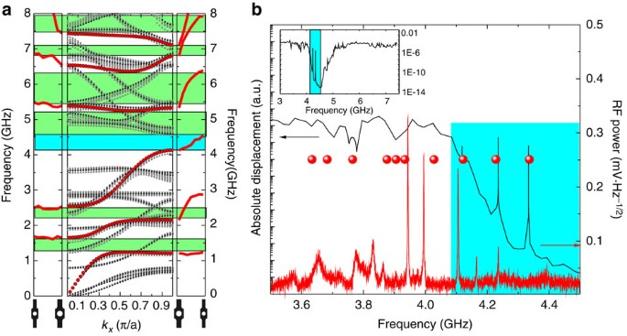Figure 4: Phononic bandgap. (a) Phononic band diagram of the mirror cells, in the central panel. Red plots: the symmetric/symmetric bands of an idealized (as designed) mirror cell. Black plots: the bands corresponding to combinations of other symmetries. Grey plots (behind the red and black ones): the simulated bands for all mirror cells as fabricated; note that the dispersion induced by the fabrication imperfections does not close the complete bandgap (coloured light blue region) or the pseudo-bandgaps (green). The lateral panels show the symmetric–symmetric confinement potentials created for the Γ (kx=0 left panel) and theX(kx=π/a right panel) symmetry points as the unit cell is varied towards the centre, including fabrication imperfections. (b) Comparison of the transmission simulated using the red contour ofFig. 1, and the RF spectroscopy measurement shown inFig. 3, zoomed around the full bandgap. The FEM simulations of the confined modes displacement are shown; they are numbered according to the corresponding peaks in the simulations (black) and the measurements (red). The value of the mechanical Q-factor also is shown. Phonon modes 1 to 3 lie in a full bandgap (light-blue region). The frequency of the confined modes found in the simulation for that range has been marked with red spheres as reference. Inset, mechanical transmission simulation, with the bandgap highlighted in light blue. Figure 4: Phononic bandgap. ( a ) Phononic band diagram of the mirror cells, in the central panel. Red plots: the symmetric/symmetric bands of an idealized (as designed) mirror cell. Black plots: the bands corresponding to combinations of other symmetries. Grey plots (behind the red and black ones): the simulated bands for all mirror cells as fabricated; note that the dispersion induced by the fabrication imperfections does not close the complete bandgap (coloured light blue region) or the pseudo-bandgaps (green). The lateral panels show the symmetric–symmetric confinement potentials created for the Γ ( k x =0 left panel) and the X ( k x =π/a right panel) symmetry points as the unit cell is varied towards the centre, including fabrication imperfections. ( b ) Comparison of the transmission simulated using the red contour of Fig. 1 , and the RF spectroscopy measurement shown in Fig. 3 , zoomed around the full bandgap. The FEM simulations of the confined modes displacement are shown; they are numbered according to the corresponding peaks in the simulations (black) and the measurements (red). The value of the mechanical Q-factor also is shown. Phonon modes 1 to 3 lie in a full bandgap (light-blue region). The frequency of the confined modes found in the simulation for that range has been marked with red spheres as reference. Inset, mechanical transmission simulation, with the bandgap highlighted in light blue. Full size image Nevertheless, the mechanical Q -factor ( Q mec = ω m · τ phon , where τ phon is the phonon decay time) measured at room temperature at atmospheric pressure is limited to values below 2,000 by intrinsic phonon scattering mechanisms, like thermo-elastic decay or Akhieser. Size effects in nanostructures change the phonon lifetime compared with bulk [37] by modifying the intrinsic scattering, that is, the thermal conductivity is strongly reduced because of diffusive boundary scattering [38] . In the regime of high frequency, extrinsic boundary scattering can become the dominant loss mechanism, when the wavelength of the phonon is comparable to the characteristic dimension of the surface roughness [37] . In summary, we designed, fabricated and measured a high- Q photonic structure capable of transducing confined phononic modes inside an absolute phononic bandgap. The confined phonons have an OM coupling ranging from the KHz to the MHz range with contributions from moving interfaces and the photoelastic effect that add constructively for many of them. Using such a cavity, we demonstrate transduction of four other family modes, confined in pseudo-gaps, up to 8 GHz. Coupling light via a tapered fibre we reach the resolved side-band limit, an self-amplification for various of these families. As discussed, the mechanical modes confined in the full bandgap are in potential a new platform for OM phonon coherent manipulation insensitive to fabrication deviations. Therefore, OM structures displaying a phononic bandgap could be disruptive in the field of cavity optomechanics. Fabrication The 1D OM crystal structures were fabricated on standard silicon-on-insulator wafers provided by SOITEC with a top silicon layer thickness of 220 nm (resistivity [ρ]: ~1–10 Ω cm −1 ; slight p-doping: ~10 15 cm −3 ) and a buried oxide layer thickness of 2 μm. The structure fabrication is based on an electron beam, direct-writing process performed on a coated 100 nm poly(methyl methacrylate) (PMMA) resist film. The electron beam exposure, performed with a Raith150 tool, was optimized to reach the required dimensions, employing an acceleration voltage of 10 keV and an aperture size of 30 μm. The PMMA is a positive resist that implies exposure of the pattern negatives (that is, of window trenches and holes). The use of such a positive resist enables creation of well-defined holes inside the waveguides and obviates the use of a second lithography process to expose resist windows for selective silica removing. Nevertheless, the use of a PMMA resist introduces certain fabrication imperfections (which could be improved by using a negative resist such as Hydrogen silsesquioxane (HSQ)) in the interfaces between wider and narrower areas comprising the overall light waveguides. After developing the PMMA resist using MIBK/IPA as developer, the resist patterns were transferred into the silicon-on-insulator samples employing an equally optimized Inductively Coupled Plasma-Reactive Ion Etching process with fluoride gases (SF6/C4F8). The two gases are injected simultaneously under typical plasma conditions for silicon etching (pressure: 20 mT, low-bias voltage, and a SF6/C4F8 flow ratio: 1.5), which produce anisotropic etching with smooth sidewalls. Once the silicon is etched, a BHF silicon oxide etch (6:1) is used to remove the 2-μm BOX-silica layer in order to release the structures. Fabrication imperfections Several imperfections are noticeable in the SEM images (see Supplementary Fig. 1 ). Rounding of the borders appears to be systematic, as the deformation of the holes into a rhombohedral form. The parallelicity of the stubs is affected by this rounding effect, and there are random variations in size and position. Dimensional and positional deviations are in the range of a few nanometres. We use the contour of the SEM images taken on the fabricated structures to model their optical and mechanical properties. Using this procedure, the imperfections are automatically incorporated in the FEM calculations, and the OM coupling rates and Q factors reported throughout this article are already limited by fabrication imperfections. Experimental methods We use a tapered silica fibre loop to couple in-coming and out-going light in the 1D OM crystal. We use the fabrication method described in ref. 39 . The tapered fibre is fabricated using a micro-heater at 1,170 °C, whereas the fibre ends are pulled at a total rate of 40 μm s −1 . A laser set to the smallest wavelength used in the experiment transmits through the fibre during fabrication. Analysis of the time-domain oscillations enables monitoring of the transition to single mode of the tapered fibre zone. After tapering the fibre, we twist it to form a stable loop of ca 30 μm of diameter ( Supplementary Fig. 2a ), which limits the contact zone between the fibre and the sample. We place the fibre in contact with the 1D OM crystal, such that it also touches a border of the sample frame, as can be seen in Fig. 2 . By regularly checking the quickly scanned optical transmission (80 nm s −1 ), we can minimize the loading that the fibre places on the 1D OM crystal. In Supplementary Fig. 3 , we show a schematic of our experimental setup. Standard transmission measurements can be done by tuning the laser wavelength in the infrared (1,460–1,600 nm) with pm accuracy. For adjusting the fibre to device position, we use a × 100 microscope objective and a CCD camera to image from above ( Fig. 2b ). The fine-tuning of the position and a coarse adjustment of the polarization are performed by manually adjusting the positioning system with sub-micrometre precision, while observing the transmission spectra in real time. For that purpose, a tunable laser (HP 8164 B system with a 81600 B laser source) is scanned over selected wavelength ranges at 80 nm s −1 scanning rate and transmission variations are collected with a slow response detector (HP 81634B). The instability of the scan laser and the signal-to-source spontaneous emission (>64 dB nm −1 ) prevent its use for RF spectroscopy. Instead, we use a more-stable laser (Nettest Tunics-BT 3648 HE 1520, signal-to-source spontaneous emission <85 dB nm −1 ). In addition, the fibre-sample system becomes unstable and self-oscillates at high powers [40] . The power is kept low for all measurements presented in the present work (<150 μW). We perform RF spectroscopy with a 12-GHz photoreciever (New Focus 1544-B) in combination with a 20-GHz Signal Analyser (Anritsu, MS2830A). Amplification of the transduced signal is obtained by using an Erbium-doped fibre amplifier (Keopsys, CEFA-C-HG-SM-50-B201-FU-FU), which improves the signal-to-noise ratio and determines the preferred wavelength range for transducing the mechanical modes. How to cite this article: Gomis-Bresco, J. et al. A one-dimensional optomechanical crystal with a complete phononic band gap. Nat. Commun. 5:4452 doi: 10.1038/ncomms5452 (2014).